Artificial synapse network on inorganic proton conductor for neuromorphic systems The basic units in our brain are neurons, and each neuron has more than 1,000 synapse connections. Synapse is the basic structure for information transfer in an ever-changing manner, and short-term plasticity allows synapses to perform critical computational functions in neural circuits. Therefore, the major challenge for the hardware implementation of neuromorphic computation is to develop artificial synapse network. Here in-plane lateral-coupled oxide-based artificial synapse network coupled by proton neurotransmitters are self-assembled on glass substrates at room-temperature. A strong lateral modulation is observed due to the proton-related electrical-double-layer effect. Short-term plasticity behaviours, including paired-pulse facilitation, dynamic filtering and spatiotemporally correlated signal processing are mimicked. Such laterally coupled oxide-based protonic/electronic hybrid artificial synapse network proposed here is interesting for building future neuromorphic systems. Human beings could easily recognize various objects and make sense out of a large amount of visual information in a complex, real world environment through a complicated computation, which is more robust, plastic and fault-tolerant than any current digital computer. Synapses dominate the architecture of the brain and are responsible for the massive parallelism, structural plasticity and robustness [1] . Synapses are the connections between the neuron circuits, and each neuron has more than 1,000 synapse connections with other neurons. As a measurement of synapse efficacy in establishing the connection between presynaptic and postsynaptic neurons, synaptic strength or synaptic weight can be precisely adjusted by the concentrations of ionic species (for example, Ca 2+ , Na + , and K + and so on) [2] , [3] , [4] Realization of physical devices with synaptic functions is of great importance for hardware implementation of the neuromorphic computation system. In the beginning, synaptic functions were emulated by complementary metal oxide semiconductor (CMOS) neuromorphic circuits, but such CMOS circuits consumed substantially more energy than a biological synapse, and it is hard to scale up the circuits to a size comparable with the brain [5] . Recently, resistive switching memory, memristors or atomic switch has been investigated in biologically inspired neuromorphic circuits [6] , [7] , [8] , [9] , [10] , [11] . Important synaptic learning rules such as spike-timing-dependent plasticity (STDP) and short-term memory to long-term memory transition have been demonstrated. In these nanoscale ionic/electronic hybrid two-terminal artificial synapses, ionic migrant/diffusion, formation of conducting filament and electrochemical reactions are very prevalent for mimicking the neural activities [7] , [10] . In biologic systems, the dendrites of a single neuron can contain hundreds to thousands of spines that typically receive inputs from synapses of axons [12] . The dendrite spine synapses not only provide an anatomical substrate for memory storage and synaptic transmission but also serve to increase the number of possible contacts between neurons. Recently, three-terminal transistors with tunable channel conductivities have been proposed for synaptic functions emulation [13] , [14] , [15] , [16] , [17] . In such synaptic transistors, voltage pulses applied on the gate electrodes are usually regarded as the presynaptic spikes or external stimuli. The channel conductance is usually regarded as synaptic weight. Then, such synaptic transistors are similar to the dendrite synapses in biologic systems. Chen et al. [16] proposed an ionic/electronic hybrid synaptic transistor by integrating an RbAg 4 I 5 ionic conductor layer and an ion-doped MEH-PPV conjugated polymer layer into the gate dielectrics. Essential synaptic dynamic functions, such as excitatory postsynaptic current (EPSC) and STDP, were successfully mimicked. More recently, oxide-based synaptic transistors gated by nanogranular SiO 2 -based proton conductor films were proposed by our group, and short-term memory to long-term memory transition behaviours were mimicked [18] . For a conventional field-effect transistor, a bottom-gate or a top-gate configuration is always adopted. 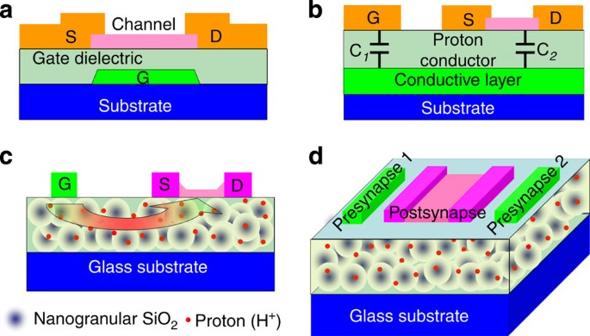Figure 1: Schematic images of transistors with different structures. (a) A traditional field-effect transistor with a bottom-gate structure. (b) An in-plane-gate transistor with a bottom conductive layer. (c) A laterally-coupled IZO transistor proposed in this work. (d) An IZO-based artificial synapse with two in-plane pre-synaptic inputs. Two in-plane gates are regarded as the presynaptic input terminals, and the self-assembled IZO channel with source/drain is regarded as the postsynaptic output terminal. Figure 1a shows a schematic image of a bottom-gate transistor, where the gate electrode is buried below the gate dielectric and the semiconductor channel. [19] , [20] . In such structure, the gate bias is coupled to the semiconductor channel through the dielectric directly. Recently, oxide-based protonic/electronic hybrid transistors with in-plane-gate configuration were invented by our group [21] , [22] , [23] , [24] . As shown in Fig. 1b , proton-conducting films, such as SiO 2 -based nanogranular films and chitosan films, were used as the gate dielectrics. Voltage applied on the in-plane-gate is coupled to the common bottom conductive layer first, and then is coupled to the channel layer, that is, the gate bias will be coupled to the channel through two gate capacitors in series. Figure 1: Schematic images of transistors with different structures. ( a ) A traditional field-effect transistor with a bottom-gate structure. ( b ) An in-plane-gate transistor with a bottom conductive layer. ( c ) A laterally-coupled IZO transistor proposed in this work. ( d ) An IZO-based artificial synapse with two in-plane pre-synaptic inputs. Two in-plane gates are regarded as the presynaptic input terminals, and the self-assembled IZO channel with source/drain is regarded as the postsynaptic output terminal. Full size image In this communication, a new type of transistor is proposed based on the proton-related lateral coupling effect. As shown in Fig. 1c , no bottom conductive layer is needed, and the gate voltage can be directly coupled to the semiconductor channel laterally by only one lateral electric-double-layer (EDL) capacitor. The indium-zinc-oxide (IZO)-based protonic/electronic hybrid transistors are self-assembled on phosphorus (P)-doped nanogranular SiO 2 proton conductive films at room temperature. Thanks to such proton-related lateral coupling effect, artificial synaptic transistor and synaptic network can be proposed, as shown in Fig. 1d . Paired-pulse facilitation (PPF), dynamic filter for information transmission and spatiotemporally correlated signal processing of biological synapse are mimicked. Such synaptic transistor network on proton conducting electrolyte film is interesting for synaptic electronics and neuromorphic systems. 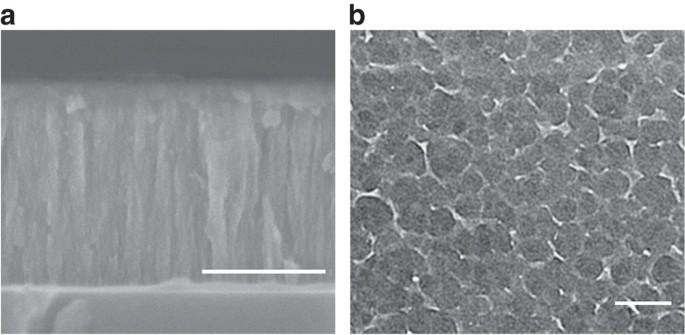Figure 2:Microstructure of the P-doped SiO2films. (a) The cross-sectional SEM image of the P-doped nanogranular SiO2electrolyte films. (Scale bar: 500 nm). (b) High-resolution TEM image of the P-doped SiO2electrolyte films on TEM Cu grid (Scale bar: 40 nm). Microstructure and electrical properties of SiO 2 films Figure 2a shows a cross-sectional scanning electron microscopy (SEM) image of the P-doped SiO 2 electrolyte films on a Si (100) substrate at room temperature. Microstructure with nanopores is observed. The thickness of the nanogranular SiO 2 films is estimated to be~820 nm. Figure 2b illustrates a high-resolution transmission electron microscope (TEM) image of the P-doped SiO 2 film deposited on TEM Cu grid at room temperature. Nanogranular SiO 2 with the size in tens of nanometre is observed. The size of the gap among the SiO 2 nanoparticles is ~2.0 nm to 5.0 nm. Therefore, high-density nanopores are formed in the electrolyte films, which provide effective channels for proton migration. Figure 2: Microstructure of the P-doped SiO 2 films. ( a ) The cross-sectional SEM image of the P-doped nanogranular SiO 2 electrolyte films. (Scale bar: 500 nm). ( b ) High-resolution TEM image of the P-doped SiO 2 electrolyte films on TEM Cu grid (Scale bar: 40 nm). Full size image Frequency-dependent specific capacitances of the P-doped nanogranular SiO 2 films were measured with a vertical IZO/SiO 2 electrolyte/indium-tin-oxide (ITO) sandwich structure ( Fig. 3a ). As shown in Fig. 3b , a large EDL capacitance >0.5 μFcm −2 can be obtained when the frequency is lower than 10 5 Hz. Such behaviors are quite similar to that measured from the ion-liquid dielectrics [25] . The capacitance curve is also measured with an in-plane structure of IZO/SiO 2 electrolyte/IZO ( Fig. 3c ). As shown in Fig. 3d , a maximum specific capacitance of ~3.0 μFcm −2 is measured at 1.0 Hz, which is due to the electric-double-layer (EDL) formation at the SiO 2 electrolyte/IZO electrode interface. Proton conductivity of the nanogranular P-doped SiO 2 film was estimated to be ~10 −4 Scm −1 at room temperature [24] . High proton conductivity is due to the sequence of proton hopping between hydroxyl groups and water molecules under applied electric field [24] , [26] , [27] . Accumulation of protons at the interface of SiO 2 electrolyte/IZO electrode will result in a large EDL capacitance and a strong lateral electrostatic coupling, which is meaningful for building artificial synaptic network [28] , [29] , [30] . The distance between the two IZO electrodes is ~300 μm. Hence, the time for proton migration to the SiO 2 electrolyte/IZO electrode interface is long, and the up-limit frequency of EDL response is low (~60 Hz). When the frequency is higher than this up-limit frequency, the measured capacitance will reduce rapidly. 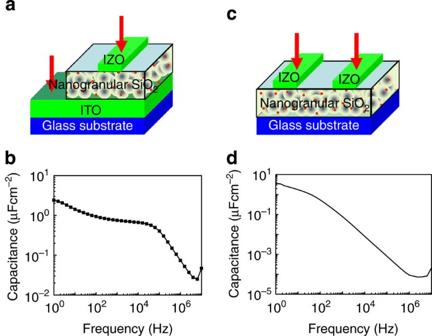Figure 3: Frequency-dependent specific capacitance. (a) A vertical sandwich structure of IZO/SiO2electrolyte/ITO. (b) Frequency-dependent specific capacitance of the P-doped SiO2electrolyte films using a vertical structure. (c) An in-plane structure of IZO/SiO2electrolyte/IZO. (d) Frequency-dependent specific capacitance of the P-doped SiO2electrolyte films with an in-plane structure. Figure 3: Frequency-dependent specific capacitance. ( a ) A vertical sandwich structure of IZO/SiO 2 electrolyte/ITO. ( b ) Frequency-dependent specific capacitance of the P-doped SiO 2 electrolyte films using a vertical structure. ( c ) An in-plane structure of IZO/SiO 2 electrolyte/IZO. ( d ) Frequency-dependent specific capacitance of the P-doped SiO 2 electrolyte films with an in-plane structure. 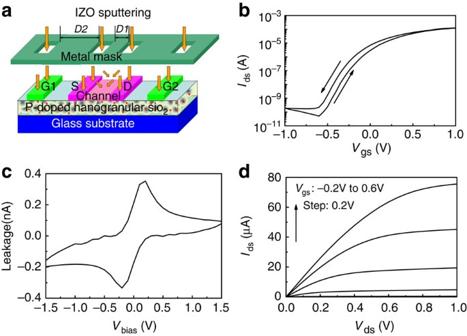Figure 4: Electrical performance of laterally coupled IZO transistor. (a) Schematic image of the self-assembled laterally coupled IZO transistor fabricated by one shadow mask method.D1=80 μm,D2=300 μm. (b) Transfer curve of the laterally-coupled IZO transistor measured atVds=1.0 V. (c) The leakage current of the SiO2electrolyte films. (d) Output curve of the laterally coupled IZO transistor. Full size image Laterally-coupled IZO transistor Figure 4a shows the schematic image of the laterally coupled IZO transistor fabricated by a one shadow mask method. When the distance between two patterns ( D1 ) is 80 μm, a thin IZO channel could be self-assembled between the IZO patterns due to the reflections of IZO nanoparticles at the mask edge and the dimensional extension of the nanoparticles with a low incident angle. When the distance between two patterns ( D2 ) is 300 μm, isolated IZO patterns can be obtained. The detail fabrication process could be found in Methods. Figure 4: Electrical performance of laterally coupled IZO transistor. ( a ) Schematic image of the self-assembled laterally coupled IZO transistor fabricated by one shadow mask method. D1 =80 μm, D2 =300 μm. ( b ) Transfer curve of the laterally-coupled IZO transistor measured at V ds =1.0 V. ( c ) The leakage current of the SiO 2 electrolyte films. ( d ) Output curve of the laterally coupled IZO transistor. Full size image The conductance of the self-assembled IZO channel between two patterned IZO films (source and drain electrodes) can be effectively modulated by another in-plane IZO pattern (gate electrode). Transfer curve ( I ds vs V gs ) of such device with a channel thickness of ~20 nm was measured with a constant V ds of 1.0 V, as shown in Fig. 4b . The gate voltage was swept from −1.0 V to 1.0 V and then back, and a clear anticlockwise hysteresis loop was observed, which is likely due to the existence of mobile protons in the nanogranular P-doped SiO 2 electrolyte [31] , [32] . The drain current on/off ratio is estimated to be ~10 6 . The leakage current of the SiO 2 electrolyte is measured to be less than 0.4 nA in the voltage range from −1.5 V to 1.5 V, as shown in Fig. 4c . Figure 4d shows a typical output curve of the laterally coupled transistor. At low V ds , drain current increases linearly with drain voltage, indicating that the device has a good ohmic contact. At higher V ds , the drain current gradually approaches to a saturated value. Such results indicate that the proposed device is a typical laterally coupled field-effect transistor. 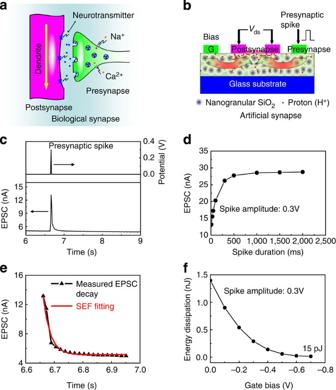Figure 5: Excitatory post-synaptic current. (a) Schematic image of a biological synapse. (b) Schematic diagram of a laterally coupled IZO synaptic transistor with two in-plane gates. (c) EPSC triggered by a presynaptic spike (0.3 V, 10 ms). EPSC is measured with aVdsof 0.5 V. (d) Spike duration-dependent EPSC, the amplitude of the spike is 0.3 V. (e) EPSC decay behaviour fitted by the stretched exponential function. (f) Energy dissipation per spike modulated by the second in-plane gate. EPSC is triggered by a presynaptic spike (0.3 V, 10 ms) and measured with aVdsof 0.5 V. Synaptic functions simulated on IZO synaptic transistor Figure 5a shows a simplified biological dendritic synapse. Synapse is the connection between two neurons in the brain, which permits a neuron to pass an electrical or chemical signal to another neuron [33] . When the in-plane gate is used as the presynaptic input terminal and the self-assembled IZO channel with source/drain electrodes is used as the postsynaptic output terminal, then an artificial synaptic transistor is proposed, as shown in Fig. 5b . A presynaptic spike applied on the in-plane-gate will trigger an excitatory post-synaptic current (EPCS) in IZO channel. Figure 5c shows a typical EPSC of the synaptic transistor with a channel thickness of ~12 nm triggered by a presynaptic spike (0.3 V, 10 ms). A V ds of 0.5 V is applied between source and drain electrode for channel EPSC measurement. The EPSC reaches a peak value of ~13 nA at the end of the spike and gradually decays back to the resting current (~5.0 nA) in ~500 ms. Such EPSC behaviour is quite similar to an EPSC process in a biological excitatory synapse [34] . The energy dissipation of single spike event is estimated to be ~45 pJ, which is lower than that of the artificial synapse based on conventional CMOS circuit [35] and is comparable to the energy dissipation of the reported hard-ware-based artificial synapse [8] , [9] , [15] . At present, the channel width of our synaptic transistors is large (~1 mm), and it can be scaled down to submicrometer scale by a photolithography method. Such scaling can further reduce the energy dissipation. Low-voltage and low-energy dissipation down to 1.0 pJ per spike is the aim for neuromorphic system application. Moreover, the energy dissipation per spike can also be reduced to ~1.0 pJ level or even sub-pJ level if the spike duration can be reduced to sub-ms level. Here, the spike duration-dependent excitatory post-synaptic currents (EPSCs) are also studied, as shown in Fig. 5d . The measured EPSC peak values increase from ~13 nA to ~29 nA for spike duration ranges from 10 ms–2,000 ms, respectively. Interestingly, the EPSC peak value increases almost linearly within a small spike duration range below ~300 ms, but it will get saturated when the spike duration is above ~300 ms. Figure 5: Excitatory post-synaptic current. ( a ) Schematic image of a biological synapse. ( b ) Schematic diagram of a laterally coupled IZO synaptic transistor with two in-plane gates. ( c ) EPSC triggered by a presynaptic spike (0.3 V, 10 ms). EPSC is measured with a V ds of 0.5 V. ( d ) Spike duration-dependent EPSC, the amplitude of the spike is 0.3 V. ( e ) EPSC decay behaviour fitted by the stretched exponential function. ( f ) Energy dissipation per spike modulated by the second in-plane gate. EPSC is triggered by a presynaptic spike (0.3 V, 10 ms) and measured with a V ds of 0.5 V. Full size image The migration of protons in the nanogranular P-doped SiO 2 film plays an important role for EPSC triggering. When a positive presynaptic spike is applied on the in-plane IZO gate, protons will migrate and accumulate at the SiO 2 /IZO channel interface, and a postsynaptic current can be measured if a small drain voltage is applied. More and more protons will migrate to the SiO 2 electrolyte/IZO channel interface when the spike duration time is increased. Hence, an increased EPSC can be obtained. However, there are only limited activated protons within the nanogranular SiO 2 matrix. Therefore, the measured EPSC in the IZO channel will become saturated at a certain spike duration time. When the spike is finished, protons will gradually drift back to their equilibrium positions. Correspondingly, the measured current in the self-assembled IZO channel will decrease gradually back to the resting current. Such proton migration-induced EPSC behaviour can be explained with the stretched exponential model and the decay of EPSC could be fitted by a stretched exponential function (SEF) [8] , [36] : where τ ˙ is the retention time, t 0 is the time when the presynaptic spike finished, I 0 is the triggered EPSC at the end of the presynaptic spike, I ∞ is the final value of the decay current and β is the stretch index ranging between 0 and 1. A good fitting curve of the decay of EPSC triggered by presynaptic spike (0.3 V, 10 ms) is obtained, as shown in Fig. 5e . τ is estimated to be ~25 ms, which means that the feature time of the protons migration is ~25 ms. To investigate the influence of voltage applied on the second in-plane-gate to the energy dissipation per spike of the synaptic transistor, synaptic transistor with dual in-plane-gate configuration is used to measure the spike-triggered EPSC. A presynaptic spike (0.3 V, 10 ms) is applied on one in-plane gate electrode, and a constant V ds of 0.5 V is used to measure the EPSC. Figure 5f shows the energy dissipation per spike modulated by the voltage applied on the second in-plane gate. When there is no bias on the second in-plane-gate (G), the energy dissipation per spike for the synaptic transistors with a channel thickness of 20 nm is ~1.4 nJ. When the voltage applied on the second in-plane-gate (G) is changed from 0 V to −0.7 V gradually, the energy dissipation gradually reduces from ~1.4 nJ to ~15 pJ. Short-term synaptic plasticity is widely believed to play an important role in synaptic computations and information processing. PPF is a phenomenon in which EPSC evoked by the spike is increased when the second spike closely follows a previous spike [37] . PPF is thus a form of short-term synaptic plasticity and was reported to be important for decode temporal information in the biological system [38] . Such PPF behaviour can also be mimicked in our synaptic transistor. 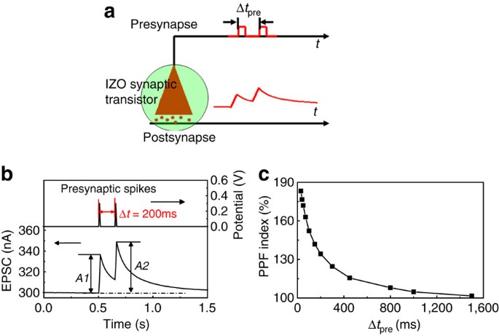Figure 6: PPF behaviors. (a) Schematic image of the excitatory postsynaptic current (EPSC). (b) A pair of presynaptic spikes and the EPSC triggered by two spikes with an inter-spike interval time of 200 ms.A1 andA2 represent the amplitudes of the first and second EPSCs, respectively. (c) PPF index, defined as the ratio ofA2/A1, plotted as a function of inter-spike interval, Δtpre, between the two consecutive pre-synaptic spikes. Figure 6a shows a schematic image of the excitatory postsynaptic current (EPSC) triggered by a pair of temporally correlated presynaptic spikes in a laterally coupled IZO-based synaptic transistor. Two consecutive presynaptic spikes (0.3 V, 10 ms) are applied on the presynapse (IZO gate) input in close succession. The inter-spike interval (Δ t pre ) ranges between 30 ms and 1,500 ms. The responses of the postsynaptic output (IZO channel) are measured in terms of EPSC at a constant V ds of 0.5 V. Figure 6b shows the EPSC triggered by the two successive presynaptic spikes with Δ t pre =200 ms. The peak value of the EPSC triggered by the second presynaptic spike is larger than that by the first presynaptic spike. The PPF index, defined as the ratio of the amplitudes between the second EPSC ( A 2) and the first EPSC ( A 1), is plotted as a function of Δ t pre in Fig. 6c . A maximum PPF index value of ~180% is obtained at Δ t pre =30 ms. When Δ t pre increases, PPF index value decreases gradually. At the end of the first spike, protons accumulated at the SiO 2 /IZO channel interface will drift gradually back to their equilibrium position due to the concentration gradient. If the second spike is applied after the first spike with a small inter-spike interval, protons triggered by the first spike still partially reside near the IZO channel. Thus, protons triggered by the second spike are augmented, which induces the PPF and short-term memory in an IZO channel. A higher PPF index value can be obtained when the applied paired spikes have a shorter Δ t pre . Figure 6: PPF behaviors. ( a ) Schematic image of the excitatory postsynaptic current (EPSC). ( b ) A pair of presynaptic spikes and the EPSC triggered by two spikes with an inter-spike interval time of 200 ms. A 1 and A 2 represent the amplitudes of the first and second EPSCs, respectively. ( c ) PPF index, defined as the ratio of A 2/ A 1, plotted as a function of inter-spike interval, Δ t pre , between the two consecutive pre-synaptic spikes. Full size image In nervous system, synaptic efficacy can increase (synaptic facilitation) or decrease (synaptic depression) markedly within milliseconds after the onset of specific temporal patterns of activity [39] . Because of the short-term synaptic depression or facilitation, synapses could also act as dynamic filters for information transmission depending on the signal frequencies [40] . The short-term synaptic depression contributes to low-pass temporal filtering and the short-term synaptic facilitation contributes to high-pass temporal filtering. Since a higher PPF index value is obtained with the shorter Δ t pre in our IZO synaptic transistor, a high-pass filter could be realized. 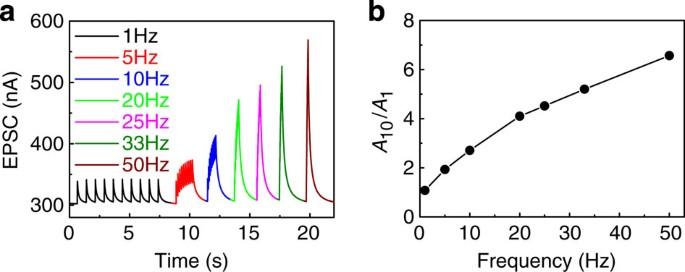Figure 7: Filter behaviors. (a) EPSCs recorded in response to the stimulus train with different frequencies. The stimulus train at each frequency consists of 10 stimulus spikes (0.5 V, 10 ms). (b) EPSCs amplitude gain (A10/A1) plotted as a function of presynaptic spike frequency. Figure 7a shows the EPSC responses of our device to the stimulus train with different frequencies. The stimulus train at each frequency consists of 10 stimulus spikes (0.3 V, 10 ms). V ds =0.5 V is applied to the source and drain electrodes for EPSCs measurements. The peak value of the EPSC keeps at ~340 nA even after 10 spikes when the frequency of the stimulus train is 1.0 Hz. When the frequency of the stimulus train is increased, the peak values of the EPSCs increase obviously. Figure 7b shows the frequency-dependent gain defined as the ratio of the amplitudes between the tenth EPSC ( A 10) and the first EPSC ( A 1). The gain increases from ~1.0 to ~6.6 when the stimulus frequency changes from 1.0 Hz to 50 Hz, which indicates that the synaptic transistor can act as the dynamic high-pass filter for information transmission. The high-pass temporal filtering mimicked here is meaningful for neuromorphic computations or artificial neural network. Figure 7: Filter behaviors. ( a ) EPSCs recorded in response to the stimulus train with different frequencies. The stimulus train at each frequency consists of 10 stimulus spikes (0.5 V, 10 ms). ( b ) EPSCs amplitude gain ( A 10/ A 1) plotted as a function of presynaptic spike frequency. Full size image The spatiotemporally correlated stimuli from different neurons will trigger a postsynaptic neuron to establish a dynamic logic. To simulate the spatiotemporal dynamic logic, laterally coupled synaptic transistor with two in-plane gates is proposed, as shown in Fig. 8a . The responses of the postsynapse are measured with a constant V ds of 0.5 V. When a presynaptic spike is applied on the pre-synapse, protons will migrate to the SiO 2 /IZO interface and trigger an EPSC. Presynaptic spike (0.5 V, 20 ms) applied on presynapse 1 will trigger an EPSC 1 with an amplitude of ~30 nA and presynaptic spike (1.0 V, 20 ms) applied on pre-synapse 2 will trigger an EPSC 2 with an amplitude of ~50 nA, as shown in Fig. 8b . When two presynaptic spikes are applied on presynapse 1 and presynapse 2, protons migrated to the interface region will be accumulated, therefore the two EPSCs will be summed in the postsynapse. Such summation is a dynamic analogue function of time and Δ t pre2−pre1 . 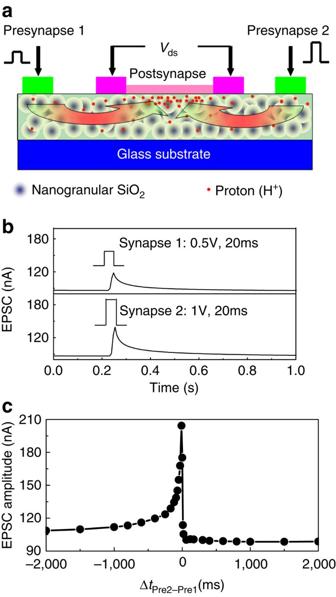Figure 8: Dynamic logic. (a) Schematic image of the laterally coupled synaptic transistor with two in-plane gates. Presynaptic spikes are applied on two in-plane IZO gates, and a constantVds=0.5 V is used to measure the EPSC. (b) EPSCs triggered by presynaptic spike 1 (0.5 V, 20 ms) and presynaptic spike 2 (1.0 V, 20 ms), respectively. (c) The amplitude of the EPSCs att=0 (when the presynaptic spike applied on the presynapse 1 finished) is plotted as a function of Δtpre2−pre1between the two presynaptic spikes. Figure 8c illustrates the amplitude of the EPSC at Δ t =0 (when the presynaptic spike applied on the Synapse 1 finished) as a function of the inter-spike interval Δ t pre2−pre1 . When Δ t pre2−pre1 =0, protons triggered by presynaptic spike 1 and presynaptic spike 2 arrive at the interface region at the same time, which means that the EPSC1 and EPSC2 are triggered simultaneously, therefore the amplitude of the EPSC in the postsynapse reaches the maximum value of ~110 nA. The summed amplitude (~110 nA) is larger than the linear sum of EPSC 1 (~30 nA) and EPSC 2 (~50 nA). The results show that the spatiotemporal EPSC summation in our laterally coupled synaptic transistor is superlinear amplification, which is similar to that observed in hippocampal CA1 pyramidal neurons [41] . When |Δ t pre2−pre1 | increases, the amplitude of the EPSC decreases asymmetrically. When the IZO presynapse 1 is triggered earlier than the IZO presynapse 2 (Δ t pre2−pre1 >0), protons triggered by presynaptic spike 2 will migrate to interface region later than that triggered by presynaptic spike 1. Thus, the amplitude of EPSC at Δ t =0 is equal to the peak amplitude of EPSC1. At the end of the presynaptic spike 2, protons accumulated at the SiO 2 /IZO channel interface will drift gradually back to their equilibrium position due to the concentration gradient. When IZO synapse 1 is triggered later than IZO Synapse 2 (Δ t pre2−pre1 <0), the protons triggered by presynaptic spike 1 will be augmented with that triggered by presynaptic spike 2. When Δ t pre2−pre1 is increased, more and more protons triggered by presynaptic spike 2 will drift back to their equilibrium position. Thus, the number of protons accumulated at the interface will decrease. Therefore, EPSC value at Δ t =0 will decrease gradually as a function of Δ t pre2−pre1 . Figure 8: Dynamic logic. ( a ) Schematic image of the laterally coupled synaptic transistor with two in-plane gates. Presynaptic spikes are applied on two in-plane IZO gates, and a constant V ds =0.5 V is used to measure the EPSC. ( b ) EPSCs triggered by presynaptic spike 1 (0.5 V, 20 ms) and presynaptic spike 2 (1.0 V, 20 ms), respectively. ( c ) The amplitude of the EPSCs at t =0 (when the presynaptic spike applied on the presynapse 1 finished) is plotted as a function of Δ t pre2−pre1 between the two presynaptic spikes. Full size image Artificial synaptic network As shown in Fig. 9a , synaptic network with multiple presynaptic inputs and multiple postsynaptic outputs can be fabricated on the proton conducting electrolyte film by a simple process. Here we should point out that all presynapses and postsynapses are all intercoupled. Hence, our laterally coupled device configuration is very interesting for synaptic network construction. Thanks to the strong lateral in-plane protonic/electronic coupling effect, no intentional hard-wire connection is needed. To check that all lateral presynapses can be coupled to the postsynapses, EPSCs stimulated by spikes from five presynapses with different distance ( d ) were measured. Presynaptic spikes (0.5 V, 10 ms) are applied on different in-plane gate electrodes and a constant V ds of 1.0 V is applied between the source/drain electrodes. As shown in Fig. 9b , a high EPSC peak value of ~630 nA is measured when d =500 μm. The EPSC peak value decreases when d is increased. When d is increased to ~3.2 mm, the measured EPSC peak value is reduced to be ~370 nA. The results obtained here suggested lateral presynapses with different d have different synaptic weights, which is interesting for synaptic network construction. Distance-dependent PPF behaviour is also studied. Two presynaptic spikes (0.3 V, 10 ms) are applied on five presynapses (IZO gates) with different distances. The inter-spike interval (Δ t pre ) is set to be 100 ms. The response of the postsynaptic (IZO channel) is measured at a constant V ds of 0.5 V. The PPF index is plotted as a function of d , as shown in Fig. 9c . A maximum PPF index value of ~143% is obtained when d =450 μm. When d is increased to ~3.2 mm, the PPF index is reduced to ~133%. Hence, our results indicate that PPF can be stimulated by all lateral presynapses, and PPF index shows a distance-dependent weight. 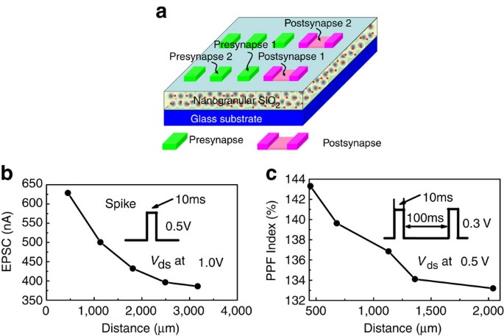Figure 9: Artificial synaptic network. (a) Schematic image of the artificial synaptic network with multiple in-plane gates (presynapses) and multiple IZO channels (postsynapses) fabricated on P-doped SiO2electrolyte films. (b) Presynapse to postsynapse distance-dependent EPSCs of the laterally coupled synaptic network. (c) The PPF index plotted as a function of the presynapse to postsynapse distance. Figure 9: Artificial synaptic network. ( a ) Schematic image of the artificial synaptic network with multiple in-plane gates (presynapses) and multiple IZO channels (postsynapses) fabricated on P-doped SiO 2 electrolyte films. ( b ) Presynapse to postsynapse distance-dependent EPSCs of the laterally coupled synaptic network. ( c ) The PPF index plotted as a function of the presynapse to postsynapse distance. Full size image Proton migration triggered by the gate pulse results in the establishments of the inter-coupling between the in-plane gates and the self-assembled IZO channels. Each lateral IZO gate and each IZO channel with IZO source/drain can be regarded as presynapse and postsynapse, respectively. In such artificial synaptic network with multiple presynaptic input terminals, the synaptic weights of the self-assembled IZO channels are spatiotemporally dependent on the spikes applied on the multiple presynaptic inputs. The synaptic arrays proposed here can be used as the building blocks for neuromorphic computations. It should be noted here that the temporal magnitude of our proposed IZO synaptic transistor is larger than that in a biology system [39] . First, the larger temporal magnitude is due to the wider spike duration time. The minimum spike duration time is 10 ms for Keithley 4200 used for our data measurement. In the future, the temporal magnitude can be improved by reducing the spike duration time down to 1.0 ms. Second, the distance between presynapse and postsynapse is in the order of 500 μm, and the time for proton migration is long. If the distance is scaled down to 10 μm, the temporal magnitude can be also greatly reduced. At last, increasing the proton conductivity of SiO 2 electrolyte can also reduce the temporal magnitude. In summary, laterally coupled IZO-based synaptic transistor network was fabricated on a nanogranular P-doped SiO 2 electrolyte film. A strong lateral electrostatic coupling effect was observed due to proton migration in the P-doped SiO 2 electrolyte film. PPF, dynamic filter function and spatiotemporal signal processing are successfully mimicked. Such oxide-based synapse network proposed here is interesting for synaptic electronics and building neuromorphic systems. Fabrication of laterally coupled IZO synaptic transistors Laterally coupled IZO synaptic transistors were fabricated on glass substrate at room temperature. First, phosphorus (P)-doped nanogranular SiO 2 films were deposited on glass substrates by plasma-enhanced chemical-vapour deposition (PECVD) using SiH 4 /PH 3 mixture (95% SiH 4 +5% PH 3 ) and O 2 as the reactive gases and Ar as plasma enhancement gas. Ratio frequency power is ~100 W and working pressure is ~30 Pa. The flow rates of the SiH 4 /PH 3 mixture (95% SiH 4 +5% PH 3 ), O 2 and Ar are 10 sccm, 60 sccm and 60 sccm, respectively. The thickness of the P-doped nanogranular SiO 2 films is ~820 nm. Then, IZO patterns were deposited on the P-doped nanogranular SiO 2 films by radio frequency magnetron sputtering IZO target in pure Ar ambient with a nickel shadow mask, as shown in Fig. 4a . Ratio frequency power, Ar flow rate and chamber pressure are 100 W, 14 sccm and 0.5 Pa, respectively. When the distance between the patterns is 80 μm, a thin IZO channel can be self-assembled between the IZO source and drain electrodes due to the reflection of IZO nanoparticles at the mask edge and dimensional extention by IZO nanoparticles with a low incident angle. The thickness of the self-assembled IZO channel layer can be controlled by the distance between metal mask and the substrate. When the distance between the patterns is as large as 300 μm, no connected channel layer can be obtained and the isolated IZO patterns are used as the in-plane gates. Microstructure characterizations of P-doped SiO 2 For microstructure characterization, P-doped SiO 2 electrolyte films were also deposited on a polished Si (100) wafers and Cu TEM grids. Field-emission scanning electron microscopy (FE-SEM, S-4800) and transmission electron microscopy (TEM, JEM-2100) were used for structural characterization of the nanogranular P-doped SiO 2 electrolyte films. Electrical measurements Proton conductivity and frequency-dependent capacitances of the P-doped SiO 2 electrolyte films were characterized by a Solartron 1260A Impedance Analyzer in air ambient with a relative humidity of ~50%. Electrical performance of the transistors and synaptic functions were measured by a semiconductor parameter characterization system (Keithley 4200 SCS) under a relative humidity of ~50%. Presynaptic spikes are applied on the in-plane gate electrodes, and post-synaptic current output is measured by applying a small reading drain voltage on the IZO source/drain electrodes. To check that all lateral presynapses can be coupled to a postsynapse, excitatory postsynaptic current (EPSC) and PPF stimulated by spikes from five presynapses were measured. How to cite this article: Zhu, L. Q. et al. Artificial synapse network on inorganic proton conductor for neuromorphic systems. Nat. Commun. 5:3158 doi: 10.1038/ncomms4158 (2014).